Electric dipoles on magnetic monopoles in spin ice The close connection of electricity and magnetism is one of the cornerstones of modern physics. This connection has a crucial role from a fundamental point of view and in practical applications, including spintronics and multiferroic materials. A breakthrough was a recent proposal that in magnetic materials called spin ice the elementary excitations have a magnetic charge and behave as magnetic monopoles. I show that, besides magnetic charge, there should be an electric dipole attached to each magnetic monopole. This opens new possibilities to study and control such monopoles using an electric field. Thus, the electric–magnetic analogy goes even further than usually assumed: whereas electrons have electric charge and magnetic dipole (spin), magnetic monopoles in spin ice, while having magnetic charge, also have an electric dipole. Spin ice materials present a very interesting class of magnetic materials [1] . Mostly these are the pyrochlores with strongly anisotropic Ising-like rare earth such as Dy or Ho [2] , although they exist in other structures, and one cannot exclude that similar materials could also be made on the basis of transition metal elements with strong anisotropy, such as Co 2+ or Fe 2+ . Spin ice systems consist of a network of corner-shared metal tetrahedra with effective ferromagnetic coupling between spins [3] , [4] , in which in the ground state the Ising spins are ordered in two-in/two-out fashion. Artificial spin ice systems with different structures have also been made [5] , [6] , [7] , [8] . Spin ice systems are bona fide examples of frustrated systems, and they attract now considerable attention, both because they are interesting in their own right and because they can model different other systems, including real water ice [9] . A new chapter in the study of spin ice was opened by the suggestion that the natural elementary excitations in spin ice materials—objects with 3-in/1-out or 1-in/3-out tetrahedra—have a magnetic charge [10] and display many properties similar to those of magnetic monopoles [11] . Especially the last proposal gave rise to a flurry of activity, see ref. 12 , in which, in particular, the close analogy between electric and magnetic phenomena was invoked. Thus, one can apply to their description many notions developed for the description of systems of charges such as electrolytes; this description proves to be very efficient for understanding many properties of spin ice. Until now the largest attention was paid to the magnetic properties of spin ice, both static and dynamic, largely connected with monopole excitations [13] , [14] , [15] , [16] , [17] , [18] , and the main tool to modify their properties was magnetic field, which couples directly to spins or to the magnetic charge of monopoles. I argue below that the magnetic monopoles in spin ice have yet another characteristic that could allow for other ways to influence and study them: each magnetic monopole, that is, the tetrahedron with 3-in/1-out or 1-in/3-out configuration, shall also have an electric dipole localized at such tetrahedron. This demonstrates once again the intrinsic interplay between magnetic and electric properties of matter. It is well known that some magnetic textures can break inversion symmetry—a necessary condition for creating electric dipoles. This lies at the heart of magnetically driven ferroelectricity in type-II multiferroics [19] . There exists, in particular, a purely electronic mechanism for creating electric dipoles. I demonstrate that a similar breaking of inversion symmetry, occurring in magnetic monopoles in spin ice, finally leads to the creation of electric dipoles on them. The appearance of dipoles on monopoles The usual description of magnetic materials with localized magnetic moments is based on the picture of strongly correlated electrons with the ground state being a Mott insulator, see ref. 20 . In the simplest cases, ignoring orbital effects and so on, one can describe this situation by the famous Hubbard model where t is the matrix element of electron hopping between neighbouring sites ij and U is the on-cite Coulomb repulsion. For one electron per site, n = N e / N =1, and strong interaction U ≫ t the electrons are localized, and there appears an antiferromagnetic nearest neighbour exchange interaction J =2 t 2 / U between localized magnetic moments thus formed (which acts together with the usual classical dipole–dipole interaction). Depending on the type of crystal lattice there may exist different types of magnetic ground state, often rather nontrivial, especially in frustrated lattices containing, for example, magnetic triangles or tetrahedra as building blocks. One can show [21] , [22] that, depending on the magnetic configuration, there can occur a spontaneous charge redistribution in such a magnetic triangle, so that for example, the electron density on site 1 belonging to the triangle (1,2,3) is (in other spin textures there may appear spontaneous orbital currents [21] , [22] in such triangles). From this expression one sees, in particular, that there should occur charge redistribution for a triangle with two spins up and one down ( Fig. 1 ), which would finally give a dipole moment shown in Fig. 1 by a broad green arrow. 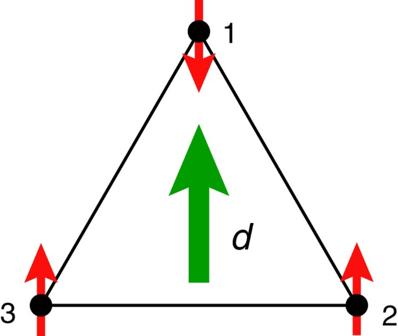Figure 1: Electronic mechanism of dipole formation. The formation of an electric dipole (green arrow) on a triangle of three spins (red arrow). Figure 1: Electronic mechanism of dipole formation. The formation of an electric dipole (green arrow) on a triangle of three spins (red arrow). Full size image A similar expression describes also an electric dipole, which can form on a triangle due to the usual magnetostriction. One can illustrate this by the example of Fig. 2 , see ref. 23 , in which we show the triangle (1,2,3) made by magnetic ions, with intermediate oxygens sitting outside the triangle and forming a certain angle M –O– M . For 3-in spins ( Fig. 2a ), all three bonds are equivalent, and all M –O– M angles are the same. However, in a configuration of Fig. 2b (which, according to equation (2), would give a non-zero dipole moment due to electronic mechanism), two bonds become 'more ferromagnetic' and the oxygens would shift as shown in Fig. 2b , so as to make the M –O– M angle in the 'antiferromagnetic' bond closer to 180°, and in 'ferromagnetic' bonds closer to 90°; according to the Goodenough–Kanamori–Anderson rules this would strengthen the corresponding antiferromagnetic and ferromagnetic exchange and lead to energy gain. As one sees from Fig. 2b , such distortions shift the centre of gravity of positive ( M ) and negative (O) charges, and thus would produce a dipole moment similar to that of Fig. 1 . A similar effect would also exist in a monopole configuration of spin ice, in which on some bonds the spins are oriented 'ferromagnetic-like' (for example, on bonds with 2-in spins), and on other bonds the spins are 'more antiferromagnetic' (bonds with 1-in and 1-out spins). 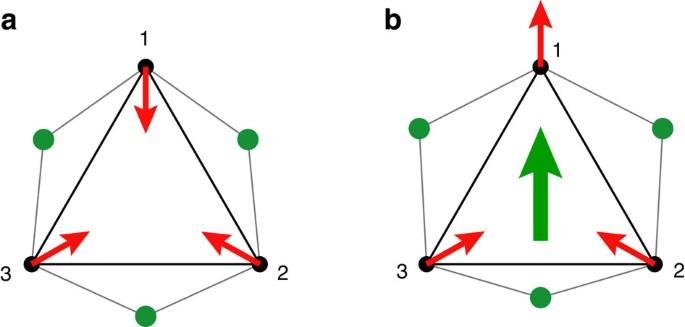Figure 2: Magnetostriction mechanism of dipole formation. Illustration of magnetostriction mechanism of the formation of an electric dipole (green arrow): the symmetric location of oxygens (green circles) for equivalent bonds (a) changes to an asymmetric one for spin configuration (red arrows) with different spin orientations on different bonds (b). Figure 2: Magnetostriction mechanism of dipole formation. Illustration of magnetostriction mechanism of the formation of an electric dipole (green arrow): the symmetric location of oxygens (green circles) for equivalent bonds ( a ) changes to an asymmetric one for spin configuration (red arrows) with different spin orientations on different bonds ( b ). Full size image The expression (3) is the main expression, which gives the 'dipole on monopole' in spin ice. Indeed, when one considers three possible configuration of a tetrahedron in spin ice, Fig. 3a (4-in or 4-out state), the basic spin ice configurations 2-in/2-out, Fig. 3b and the monopole configuration of Fig. 3c,d , then, applying the equations (2), (3) to every triangle constituting a tetrahedron, one can easily see that there would be no net dipole moments in the cases of Fig. 3a (4-in or 4-out) and Fig. 3b (2-in/2-out), but there will appear a finite dipole moment in the case of Fig. 3c,d , that is, there will appear an electric dipole on each magnetic monopole in spin ice. 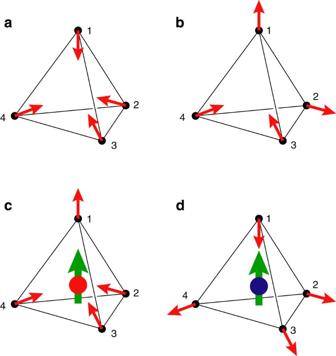Figure 3: Formation of dipoles on monopoles. Possible spin states (red arrows) in spin-ice-like systems, showing the formation of electric dipoles (broad green arrow) in monopole and antimonopole configurations. Dipoles are absent in 4-in (a) and 2-in/2-out (b) states, but appear on the monopole (c) and antimonopole (d). Note that the direction of dipoles in cases (c,d) is the same (in the direction of the 'special' spinS1). Figure 3: Formation of dipoles on monopoles. Possible spin states (red arrows) in spin-ice-like systems, showing the formation of electric dipoles (broad green arrow) in monopole and antimonopole configurations. Dipoles are absent in 4-in ( a ) and 2-in/2-out ( b ) states, but appear on the monopole ( c ) and antimonopole ( d ). Note that the direction of dipoles in cases ( c , d ) is the same (in the direction of the 'special' spin S 1 ). Full size image The easiest way to check this is to start from the case of Fig. 3a , with 4-in spins. The total charge transfer, for example, on site 1 is For the 4-in state, all the scalar products ( S i · S j ) are equal, that is, the charge redistribution, and with it the net dipole moment of the tetrahedron is zero. (One can also use the condition S 1 + S 2 + S 3 + S 4 =0, valid in this case, to prove this; the fact that the dipole moment is zero also follows just from the symmetry). However, when we reverse the direction of one spin, for example, S 1 →− S 1 , creating a 3-in/1-out monopole configuration of Fig. 3c , the first term in equation (4) changes sign, and the resulting charge transfer from sites 2, 3 and 4 to site 1 would be non-zero—and there will appear a dipole moment on such a tetrahedron, directed from the centre of the tetrahedron to the site with the 'special spin', in this case to site 1—the broad green arrow in Fig. 3c (or in the opposite direction, depending on the specific situation—the sign of the hopping t in equation (2), or the details of the exchange striction). This conclusion, shown in Fig. 3c,d , is actually the main result of this paper. As the expressions (2)–(4) for the charge redistribution and for the dipole moment are even functions of spins S , the reversal of all spins will not change the results. Thus, the magnitude and the direction of the electric dipole is the same for both the monopole (3-in/1-out) and antimonopole (1-in/3-out) configurations, Fig. 3c,d : in both cases the dipole points in the direction of the 'special' spin. Similar considerations show that when we change the direction of one more spin, for example, S 2 →− S 2 , creating the 2-in/2-out configuration of Fig. 3b , various terms in equation (4) again cancel, and such spin configurations do not produce electric dipole. Thus, electric dipoles appear in spin ice only on monopoles and antimonopoles. Some consequences The appearance of electric dipoles on monopoles in spin ice could have many consequences, some of which we now discuss. The main effect would be the coupling of such dipoles to the DC or AC electric field, This would give an electric activity to monopoles, allow one to influence them by external electric field and would thus open a new way to study and control such monopoles in spin ice. Because of this coupling, the monopoles would contribute to the dielectric function ( ω ). Actually such effect was observed in ref. 24 , where it was found that the dielectric function has strong anomalies in Dy 2 Ti 2 O 7 in the magnetic field in the [111] direction when the system approaches a transition to the saturated state at H ~1 T [25] ]. The mechanism of these anomalies was not discussed in ref. 24 , but one can connect it with the proliferation of monopoles and antimonopoles, with the corresponding electric dipoles on each of them, in approaching this transition. The saturated state in this situation, shown in Fig. 4 , has the form of staggered monopoles–antimonopoles at every tetrahedron. From our results presented above, we conclude that in this state there would also be electric dipoles at every tetrahedron, shown in Fig. 4 by thick green arrows. We see thus that this saturated state in a strong enough [111] magnetic field would simultaneously be antiferroelectric. Thus, one can also associate the anomalies observed in ref. 24 in ( ω ) in approaching this state as the anomalies at the antiferroelectric transition. 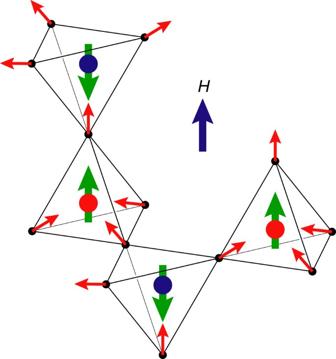Figure 4: Ordered spin configuration in spin ice in a strong [111] magnetic field. This structure can be seen as an ordered array of monopoles and antimonopoles; simultaneously it is antiferroelectric (electric dipoles are shown by broad green arrows). Figure 4: Ordered spin configuration in spin ice in a strong [111] magnetic field. This structure can be seen as an ordered array of monopoles and antimonopoles; simultaneously it is antiferroelectric (electric dipoles are shown by broad green arrows). Full size image Yet another consequence of the appearance of dipoles on monopoles could be the possibility of changing the activation energy for creating such monopoles by electric field: the excitation energy of a monopole, or the monopole–antimonopole pair would be Correspondingly, depending on the relative orientation of d and E , the excitation energy can both increase and decrease, but one can always find configurations of monopoles for which the energy would decrease. One should then be able to see this change of activation energy in thermodynamic and magnetic properties, such as specific heat and so on. The orientation of electric dipoles depends on the particular situation. One can easily see that in the absence of magnetic fields, for completely 'free', random spin ice, in general the orientation of dipoles on monopole excitations is random, in all [111] directions. But, for example, in strong enough [001] magnetic field, in which the spin ice state is ordered ( Fig. 5 ), the monopoles and antimonopoles would have the z components of dipoles, respectively, positive and negative, d z (monopoles)>0, d z (antimonopoles)<0 , whereas the perpendicular projections of d would be random. Similarly, in the [110] field [26] , the xy -projection of dipole moments will be parallel to the field, d xy ||[110]. 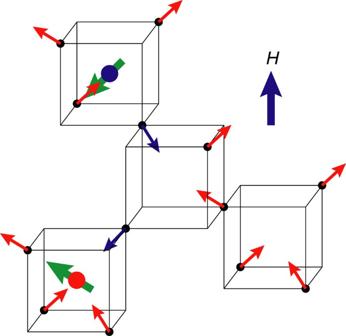Figure 5: Possible monopole–antimonopole pair in strong [001] magnetic field. Thezcomponent of electric dipoles (broad green arrows) on monopoles is pointing up, and on antimonopoles down. The perpendicular components ofdpoint in random [110] and [1[macr1]0] directions. Blue arrows show spins inverted in creating and moving apart monopole and antimonopole. Figure 5: Possible monopole–antimonopole pair in strong [001] magnetic field. The z component of electric dipoles (broad green arrows) on monopoles is pointing up, and on antimonopoles down. The perpendicular components of d point in random [110] and [1[macr1]0] directions. Blue arrows show spins inverted in creating and moving apart monopole and antimonopole. Full size image Yet another effect could appear in an inhomogeneous electric field, created for example close to a tip with electric voltage applied to it, in an experimental set-up shown in Fig. 6 (as, for instance, in the study of Néel domain walls in a ferromagnet, which also develop electric polarization and which can be influenced by inhomogeneous electric field [27] ). As always, the electric dipoles would move in grad E , with positive dipoles for example being attracted to the region of stronger field and negative ones repelled from it. One can use this effect to 'separate' monopoles from antimonopoles. Thus, as is clear from Fig. 4 , in a [111] magnetic field, such as in the phase of 'kagome ice' [25] , the 'favourable' monopoles would have dipole moments up, and antimonopoles down, so that the monopoles would be attracted to the tip, to the region of stronger electric field, and antimonopoles would be repelled from the tip. Similarly, the monopole–antimonopole separation could be reached in a [001] magnetic field, in which, as we have argued above ( Fig. 5 ), monopoles have d z >0, and antimonopoles have d z <0. 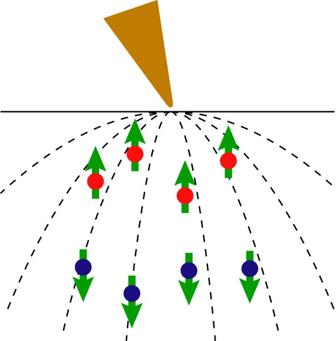Figure 6: Separation of monopoles and antimonopoles. The behaviour of monopoles and antimonopoles with respective electric dipoles (green arrows) in spin ice in [111] or [001] magnetic field in the inhomogeneous electric field (dashed lines) created by a tip (brown) with electric voltage. Figure 6: Separation of monopoles and antimonopoles. The behaviour of monopoles and antimonopoles with respective electric dipoles (green arrows) in spin ice in [111] or [001] magnetic field in the inhomogeneous electric field (dashed lines) created by a tip (brown) with electric voltage. Full size image The magnitude of the dipoles created on monopoles, and the corresponding strengths of their interaction with electric field, depend on the detailed mechanism of their creation and on the specific properties of a given material. One should think that in real spin ice materials, in which the hopping of f electrons is rather small, it is the magnetostriction mechanism of the dipole formation on monopoles and antimonopoles that would be the dominant one. In this case, one could make a crude estimate based on the interaction (5). If the shifts of ions u due to striction would be for example of order 0.01 Å, then the change of the energy =− d · E=−d·E=−euE in a field E ~10 5 V cm −1 would be ~0.1 K—which would lead to measurable effects, as the typical excitation energy of monopoles in spin ice is ~0.1 K [1] , [11] . We would get effects of the same order of magnitude for the distortions u ~10 −3 Å in a field ~10 6 V cm −1 . Summarizing, I have demonstrated that there should appear real electric dipoles on magnetic monopoles in spin ice. Creation of such dipoles may lead to many experimental consequences, some of which were discussed above. They can open new ways to study and to manipulate these exciting new objects—magnetic monopoles in a solid. We also see that the close connection between electric and magnetic phenomena, which lies at the heart of modern physics, extends in this case even further than one thought: in these systems one can have not only magnetic charges instead of electric ones, and 'magnetricity' instead of electricity, but also similar to electrons, which have electric charge and magnetic dipole (spin), magnetic monopoles in spin ice will have magnetic charge and electric dipole. How to cite this article: Khomskii, D. I. Electric dipoles on magnetic monopoles in spin ice. Nat. Commun. 3:904 doi: 10.1038/ncomms1904 (2012).